Structure of the Acid-sensing ion channel 1 in complex with the gating modifier Psalmotoxin 1 Venom-derived peptide toxins can modify the gating characteristics of excitatory channels in neurons. How they bind and interfere with the flow of ions without directly blocking the ion permeation pathway remains elusive. Here we report the crystal structure of the trimeric chicken Acid-sensing ion channel 1 in complex with the highly selective gating modifier Psalmotoxin 1 at 3.0 Å resolution. The structure reveals the molecular interactions of three toxin molecules binding at the proton-sensitive acidic pockets of Acid-sensing ion channel 1 and electron density consistent with a cation trapped in the central vestibule above the ion pathway. A hydrophobic patch and a basic cluster are the key structural elements of Psalmotoxin 1 binding, locking two separate regulatory regions in their relative, desensitized-like arrangement. Our results provide a general concept for gating modifier toxin binding suggesting that both surface motifs are required to modify the gating characteristics of an ion channel. Acid-sensing ion channels (ASICs) are proton-gated ion channels of the Degenerin/Epithelial sodium channel family (Deg/ENaC) and function as sodium-selective pores in the nervous system of vertebrates [1] , [2] . Among the ASICs, ASIC1 channels are responsible for transient, H + -evoked currents in neurons of the central nervous system and are involved in the physiological processes of learning and sensory perception such as pain [3] , [4] . Moreover, high levels of ASIC1 are located in the amygdala of mice suggesting a contribution to behavioural disorders including anxiety and depression [5] , [6] , [7] . The minimal functional unit of ASIC1 and P2X receptors, and likely other members of the Deg/ENaC family, is a trimer in cellular membranes comprising a large extracellular body and a transmembrane-spanning pore [8] , [9] , [10] , [11] , [12] . X-ray structures of ASIC1 indicate that the primary sites for proton binding are located in three deep acidic pockets of the extracellular domains [9] , [10] . Residues from adjacent subunits form these putative pH sensors including the palm region, which contains the central and extracellular vestibule, and the cysteine-rich thumb region, which moves on acidification to open the ion pathway ( Supplementary Fig. S1 ). The ion pore is formed by six transmembrane helices of which the three carboxy-terminal helices provide the residues that act as a selectivity filter [10] and determine the pore size in the open and closed state [13] . The decrease of extracellular pH triggers the conductance of sodium ions across the lipid bilayer until desensitization [14] , [15] . On prolonged exposure to a pH of around 7.2, ASIC1 undergoes steady-state desensitization and becomes unavailable for activation and sodium conduction. ASIC1-evoked currents can be inhibited by small unspecific modulators such as amiloride or the amidine A-317567 (refs. 16 , 17 ). In contrast, selective and potent modulation of ASIC1 has so far only been observed for the agonizing heteromeric Texas coral snake toxin MitTx [18] , or the inhibitory cysteine knot toxin Psalmotoxin1 (PcTx1), from the venom of the tarantula Psalmopoeus cambridgei [19] , [20] , [21] , [22] . PcTx1 has an analgesic effect in rodent models of acute pain and provides neuroprotection in a mouse model of ischemic stroke [4] , [23] . It exclusively interacts with the homotrimeric assembly of ASIC1 in the extracellular domain and interferes with channel opening and gating [24] . On binding, a significant shift of the activation and desensitization curve to more basic pH was reported [24] , [25] , [26] . The location of PcTx1 binding was identified in the cysteine-rich region of the extracellular domain by electrophysiological and radioligand binding studies on ASIC chimeras [22] . Because the molecular interactions at the interface have not been experimentally determined, several in silico studies have attempted to dock solution NMR structures of PcTx1 (refs 27 , 28 , 29 ) onto the apo crystal structure of chicken ASIC1 (ref. 9 ). PcTx1 displays a combination of positive charge, previously postulated to be important for ASIC1 binding, and a hydrophobic region [21] . Although evidence exists that Psalmotoxin 1 acts as a gating modifier [21] , [24] , it has so far not been included in the well-characterized family of gating modifier toxins such as Hanatoxin or VSTx1 that modify voltage-gated ion channels [30] . Despite their structural diversity, all these gating modifier toxins feature a hydrophobic patch and a basic cluster. Sequence alignments and mutagenesis studies suggest that residues in the S3–S4 linker region of voltage-gated ion channels are important for binding but a clear picture of how gating modifier toxins bind remains unclear [30] . The goal of this present study was to understand the molecular mechanism of PcTx1 binding and modulation of the ASIC1. We established patch clamp and surface plasmon resonance assays to demonstrate that PcTx1 binds to isolated, detergent solubilized ASIC1 with characteristics similar to ASIC1 in cellular membranes. We co-purified and crystallized the chicken PcTx1-ΔASIC1 complex to determine the structure of the gating modifier toxin ligand-gated ion channel complex. Our results show the binding mode of PcTx1 to ASIC1 and allow us to propose a general concept for binding and modulation that might be applicable to all members of the gating modifier toxin family. PcTx1 binding to cellular and solubilized ASIC1 channels For the analysis of the binding properties of synthetic PcTx1, we used chicken and human ASIC1 variants expressed in Sf9 cells. In our electrophysiological experiments, wild-type human ASIC1 exhibits the characteristic pH-dependent-activation curve and shows a decrease of the measured sodium currents in the presence of 1 nM and 10 nM PcTx1 of 51% and 92%, respectively ( Supplementary Fig. S2 ). We established a surface plasmon resonance (SPR) direct binding assay to show that engineered, solubilized non-conducting versions of ASIC1 (ref. 9 ) keep the PcTx1 binding properties of the physiologically active channel. In our SPR experiments, purified minimally functional human ASIC1(1-467), human ASIC1(25-464) and the crystallized chicken ΔASIC1(26-463) bind PcTx1 with a K D of ~2 nM ( Fig. 1a ). The slow association and dissociation rates observed by SPR are similar to those reported for two-electrode voltage clamp experiments [24] and suggest that the PcTx1 binding sites of purified, truncated ASIC1 and of functional channels in cells are equivalent ( Supplementary Table S1 ). In addition, a one-to-one binding model fits the experimental SPR data indicating that a single population of PcTx1 binding sites exists in the homotrimer. These binding sites differ from that of small molecule inhibitors such as A-317567. In SPR competition binding experiments, we demonstrate that PcTx1 and A-317567 can interact simultaneously with the channel and therefore address separate binding sites ( Supplementary Fig. S3a ). 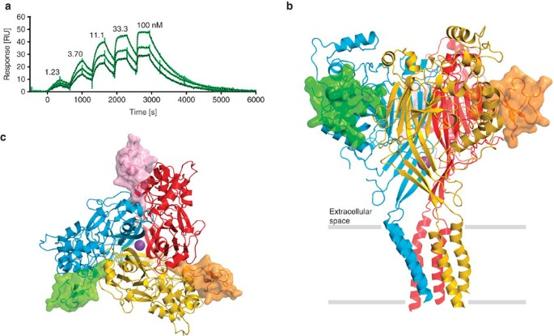Figure 1: PcTx1–ASIC1 structure and function. (a) SPR direct binding measurement42of the interaction of PcTx1 with ASIC1 channels. Green lines depict the SPR response data from a series of PcTx1 concentrations on biotinylated human ASIC1(1-467, top), human ASIC1(residues 25-464, middle) and chicken ASIC1(26-463, bottom) immobilized on a streptavidin coated chip. Black dashed lines indicate the excellent calculated fit of the SPR binding curves using a mathematical one-to-one interaction model. The virtually identical kinetics and binding constants (kon,koffandKD) indicate that PcTx1 binds equally well with an affinity of about 2 nM to the crystallized chicken ASIC1 variant and to electrophysiological functional human ASIC1. (b) Side view of the PcTx1–ASIC1 complex in ribbon representation with the sodium channel subunits in yellow, blue and red and the individual PcTx1 molecules in orange, green and purple. PcTx1 polypeptides are emphasized by transparent surface representation and are bound 50 Å above the membrane at the extracellular domains of ASIC. A putative trapped ion, at the centre of the extracellular domains, is indicated by a purple sphere. The grey lines depict the position of the lipid bilayer based on the hydrophobicity of the protein surface. (c) View from the extracellular space, perpendicular to the membrane and along the three-fold molecular and non-crystallographic symmetry axis. The three PcTx1 molecules bind between adjacent subunits of the ASIC1 homotrimer. Figure 1: PcTx1–ASIC1 structure and function. ( a ) SPR direct binding measurement [42] of the interaction of PcTx1 with ASIC1 channels. Green lines depict the SPR response data from a series of PcTx1 concentrations on biotinylated human ASIC1(1-467, top), human ASIC1(residues 25-464, middle) and chicken ASIC1(26-463, bottom) immobilized on a streptavidin coated chip. Black dashed lines indicate the excellent calculated fit of the SPR binding curves using a mathematical one-to-one interaction model. The virtually identical kinetics and binding constants ( k on , k off and K D ) indicate that PcTx1 binds equally well with an affinity of about 2 nM to the crystallized chicken ASIC1 variant and to electrophysiological functional human ASIC1. ( b ) Side view of the PcTx1–ASIC1 complex in ribbon representation with the sodium channel subunits in yellow, blue and red and the individual PcTx1 molecules in orange, green and purple. PcTx1 polypeptides are emphasized by transparent surface representation and are bound 50 Å above the membrane at the extracellular domains of ASIC. A putative trapped ion, at the centre of the extracellular domains, is indicated by a purple sphere. The grey lines depict the position of the lipid bilayer based on the hydrophobicity of the protein surface. ( c ) View from the extracellular space, perpendicular to the membrane and along the three-fold molecular and non-crystallographic symmetry axis. The three PcTx1 molecules bind between adjacent subunits of the ASIC1 homotrimer. Full size image Complex structure and molecular interactions To analyse the molecular interaction between PcTx1 and chicken ΔASIC1(26-463), we co-purified the complex and determined the crystal structure at 3.0 Å resolution ( Fig. 1b,c ; Supplementary Fig. S3b,c and Supplementary Table S2 ). In the complex, the trimeric extracellular assembly adopts the conformation known from the apo ASIC1 structures, and features the central vestibule and the ion inlet windows of the extracellular vestibule above the pore [9] , [10] . This conformation was previously assigned to the closed, desensitized-like state [9] . Three PcTx1 molecules per ASIC1 trimer are bound at the acidic pockets of the extracellular domain at the interfaces of two subunits about 50 Å above the membrane ( Fig. 2a ). The location and conformation of the carboxylate pairs Asp238-Asp350, Glu239-Asp346 and Glu220-Asp408 implicated in proton-sensing are conserved in both the apo and the complex structure. 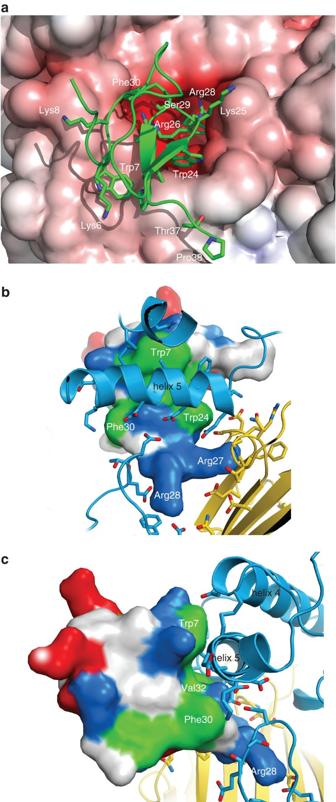Figure 2: PcTx1 binding at the acidic pockets. (a) Electrostatic surface potential representation of the acidic pocket of ASIC1 with bound PcTx1 in green ribbon representation. Contours are from −12 (red) to +12 kT (blue) through 0 (white). Side chains of PcTx1 residues relevant for the interaction are shown. (b) Surface representation of PcTx1 viewed from the bottom of the acidic pocket of ASIC1 in ribbon representation with the subunits in yellow and blue. The hydrophobic patch of PcTx1 wraps around helix 5 of ASIC1 and shields from bulk solvent the basic cluster that extends deeply into the acidic pocket. Acidic residues (Asp, Glu) of PcTx1 are depicted in red, basic residues (Arg, Lys) in blue and hydrophobic residues (Trp, Phe, Val) in green. (c) View along helix 5 at the surface of ASIC1. Figure 2: PcTx1 binding at the acidic pockets. ( a ) Electrostatic surface potential representation of the acidic pocket of ASIC1 with bound PcTx1 in green ribbon representation. Contours are from −12 (red) to +12 kT (blue) through 0 (white). Side chains of PcTx1 residues relevant for the interaction are shown. ( b ) Surface representation of PcTx1 viewed from the bottom of the acidic pocket of ASIC1 in ribbon representation with the subunits in yellow and blue. The hydrophobic patch of PcTx1 wraps around helix 5 of ASIC1 and shields from bulk solvent the basic cluster that extends deeply into the acidic pocket. Acidic residues (Asp, Glu) of PcTx1 are depicted in red, basic residues (Arg, Lys) in blue and hydrophobic residues (Trp, Phe, Val) in green. ( c ) View along helix 5 at the surface of ASIC1. Full size image All three PcTx1 molecules exhibit the same binding mode using a hydrophobic patch and a basic cluster for interaction with ASIC1 ( Fig. 2b,c ). The hydrophobic patch provides the residues Trp24, Trp7, Phe30, Val32, Val34, Pro35 and the nonpolar part of the Lys6, Lys8 and Arg26 side chains that wrap around helix 5 at the surface of the thumb. The basic cluster is dominated by Arg27 and Arg28 that extend deeply into the acidic pocket and contact the palm. The toxin locks the relative arrangement between thumb and palm in the desensitized state. The hydrophobic patch of PcTx1 interacts primarily with Phe351, Pro347, Asn321, Ala348 and with the aliphatic parts of the side chains of Glu343, Asp350, Lys342 and Lys355 in helix 5 ( Fig. 3a,b and Table 1 ). 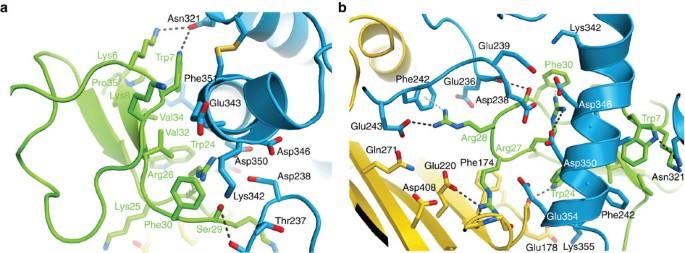Figure 3: Molecular interactions at the interface. (a) Ribbon representation of PcTx1 (green) and two of the three ASIC1 subunits (yellow and blue) viewed along helix 5 of the thumb at the surface of the extracellular domain. Side chains of residues with an intermolecular distance of ≤5 Å are shown detailing the interaction of the hydrophobic patch of PcTx1 with helix 5 of ASIC1. (b) View from the bottom of the acidic pocket outwards to the extracellular space. The view describes the charge–charge interactions between arginines of the basic cluster and the proton-sensing glutamates and aspartates of the ASIC1 palm, thumb and ball. The ASIC1 residues observed to interact with PcTx1 belong to the construction domains 3, 4 and 5 required for PcTx1 binding in ASIC1 chimeras22. Figure 3: Molecular interactions at the interface. ( a ) Ribbon representation of PcTx1 (green) and two of the three ASIC1 subunits (yellow and blue) viewed along helix 5 of the thumb at the surface of the extracellular domain. Side chains of residues with an intermolecular distance of ≤5 Å are shown detailing the interaction of the hydrophobic patch of PcTx1 with helix 5 of ASIC1. ( b ) View from the bottom of the acidic pocket outwards to the extracellular space. The view describes the charge–charge interactions between arginines of the basic cluster and the proton-sensing glutamates and aspartates of the ASIC1 palm, thumb and ball. The ASIC1 residues observed to interact with PcTx1 belong to the construction domains 3, 4 and 5 required for PcTx1 binding in ASIC1 chimeras [22] . Full size image Table 1 Summary of interactions between PcTx1 and the two subunits of trimeric chicken ASIC1 that PcTx1 contacts. Full size table The residues of the basic cluster that are flexible in solution [20] , [21] engage in a multitude of interactions and adopt a defined conformation in the complex. The guanidinium group of Arg27 forms H-bonds with the backbone carbonyls of Thr215 and Gly216 and the carboxylate of Glu220 (palm). It is located 4.5 Å away from the carboxylate of Glu354 (helix 5) of the neighbouring subunit close enough to form an electrostatic interaction. Additional nonpolar interactions of Arg27 are visible with Phe174, Phe175, Asn217, Gly218 and Glu220. Arg28 of PcTx1 penetrates the pocket the most, forms H-bonds with the carboxylate of Glu243 and is involved in a cation-π interaction with Phe242. It provides additional nonpolar interactions with some of the loop-residues between β-strands 6 and 7. Arg26 is not involved in H-bond formation to ASIC1 but its intramolecular cation-π interaction with Phe30 and the H-bond to Ser29 stabilize the PcTx1 conformation. Ser29 of PcTx1 forms an H-bond with the carbonyl group of Glu236 of the channel. Lys6 and Trp7 form H-bonds with the amide of Asn321 in helix 4 (thumb). The remaining basic and acidic PcTx1 residues are not involved in intermolecular interactions and constitute the solvent accessible surface of PcTx1 at the far side. Extra electron density in the central vestibule To understand the effect of PcTx1 binding on ASIC1, we further analysed the complex structure and found unallocated electron density in the extracellular domain. Strikingly, the electron density was visible in the occluded, central vestibule about 20 Å above the ion-selective pore. Residues from all three subunits contribute to the inner surface of the vestibule. In the desensitized-like conformation, the hydrophobic residues Leu78 and Ile419 form an obstruction at the bottom and shield the central vestibule from the extracellular vestibule that is accessible for ions ( Fig. 4a ). It was previously suggested that the central vestibule functions as a cation reservoir [10] , [31] , [32] based on the observation that mostly acidic residues line the vestibule including Glu374, Glu412, Gln277, Gln279 as well as Glu80 and Glu417. The observed extra electron density is located near Glu80 and Glu417. The carboxylate groups of Glu417 seem to coordinate a cation right above Leu78 that separates the central from the extracellular vestibule ( Fig. 4b ). Arg370 that is conserved in P2X receptors is the only positively charged residue in the central vestibule and located about 7.5 Å above the putative cation. Except for a shift of helices 4 and 5 of the thumb of ~1.3 Å towards the toxin, we cannot identify other significant changes in the extracellular domain. 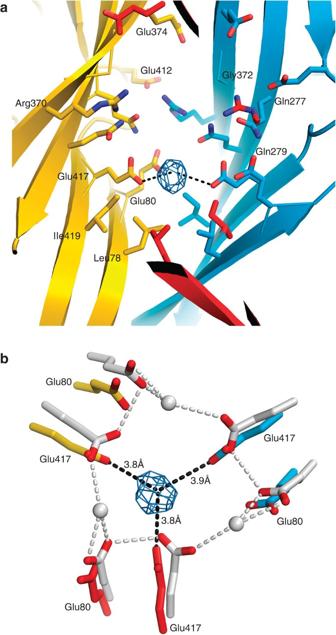Figure 4: Cation-binding site in the central vestibule. Ribbon representation of the PcTx1–ASIC1 complex with the sodium channel subunits in blue, yellow and red. (a) The complex structure in side view is sliced open at the front to provide a view inside the occluded, central vestibule highlighting some of its residues at the inner surface in stick representation. The location of the ion is indicated by the observed electron density (blue mesh) bound at position Glu417 right above Leu78 that shields the occluded vestibule from ion entrance at the extracellular vestibule. (b) Superposition and top view of the apo ASIC1 structure at 1.9 Å in white and the PcTx1 complex structure. The view reveals the electron density of the putative cation (blue mesh) bound at position Glu417 in the complex structure. In the apo ASIC1, the carboxylate groups of Glu417 are rotated to coordinate water molecules and form intrasubunit H-bonds with Glu80. Figure 4: Cation-binding site in the central vestibule. Ribbon representation of the PcTx1–ASIC1 complex with the sodium channel subunits in blue, yellow and red. ( a ) The complex structure in side view is sliced open at the front to provide a view inside the occluded, central vestibule highlighting some of its residues at the inner surface in stick representation. The location of the ion is indicated by the observed electron density (blue mesh) bound at position Glu417 right above Leu78 that shields the occluded vestibule from ion entrance at the extracellular vestibule. ( b ) Superposition and top view of the apo ASIC1 structure at 1.9 Å in white and the PcTx1 complex structure. The view reveals the electron density of the putative cation (blue mesh) bound at position Glu417 in the complex structure. In the apo ASIC1, the carboxylate groups of Glu417 are rotated to coordinate water molecules and form intrasubunit H-bonds with Glu80. Full size image Our study on the PcTx1–ASIC1 complex describes, to our knowledge, the first three-dimensional structure of a gating modifier toxin bound to an ion channel. The experimental data shows that maximally three toxin molecules can bind to one ASIC1 trimer and provides the molecular interactions at the PcTx1–ASIC1 interface. We infer a concept of bimodal binding and motion restriction of regulatory regions for the gating modifier Psalmotoxin 1 that may be common for all gating modifier toxins such as Hanatoxin and VSTx1 inhibiting voltage-gated potassium channels [30] , [33] , [34] , [35] . These gating modifier toxins have an amphipathic nature and possess hydrophobic and charged surface regions [30] . PcTx1 shares the same surface motifs ( Supplementary Fig. S4 ). The PcTx1–ASIC1 complex structure illustrates that these two surface motifs are required for channel binding and modulation ( Fig. 2b,c ). PcTx1 uses the hydrophobic patch to bind to the thumb region of the ASIC1 channel and the basic cluster to extend into the ligand-binding site and establish strong interactions by forming H-bonds. The thumb is implied in moving the transmembrane helices and the palm features the ion inlet windows and cation reservoir. PcTx1 can interact with ASIC1 in the open conformation but it seems to eventually stabilize the desensitized state [25] . By binding simultaneously to both the thumb and the palm of adjacent subunits, it locks the two regulatory regions in their relative, desensitized-like arrangement. This makes ASIC1 unavailable for further activation neither by protons nor by agonists such as MitTx [18] . Although the structures of gating modifier toxins and the effect on the individual ion channels may vary from case to case, we conclude that such bimodal binding is needed to cause the modulation. In voltage-gated ion channels, besides the interaction with residues in the S3–S4 linker region [36] , additional regions likely contribute to gating modifier toxin binding. It remains to be seen if lipids have a role for toxin binding to voltage-gated channels, however, it is evident from the crystal structure that no lipids are involved at the PcTx1–ASIC1 binding interface. Although we reason that both surface motifs are key structural elements of gating modification, the hydrophobic patch has a major role for the interaction and additionally amplifies the charge-related interactions between the basic cluster and the carboxylates in the acidic pocket. For small molecules, the single best structural parameter correlating with the binding affinity is the amount of hydrophobic surface buried on ligand binding, whereas hydrogen bonds typically convey specificity to a recognition process [37] . Hydrogen bonds do not necessarily add free energy for binding. At protein–protein interfaces, the hydrophobic effect is not the only but typically the dominating parameter complex [38] . And indeed the biggest part of the binding surface is made up by hydrophobic interactions in the PcTx1–ASIC1 complex. Importantly, the extensive hydrophobic surface surrounds the positively charged guanidinium groups of the arginines in the basic cluster. This hydrophobic seal enhances the electrostatic contribution of their charge–charge interactions with ASIC1 carboxylates by shielding the charges from the bulk water in the complex similar to the hydrophobic O-rings located around binding hot spots, typically observed at protein–protein interfaces ( Fig. 2b,c ) [39] . The use of a structural alignment of ASIC channels and the analysis of the binding interface explains why PcTx1 is surprisingly selective for ASIC1 despite the high sequence similarity among ASIC channels. Of around 30 chicken ASIC1 residues with a distance of less than 5 Å to PcTx1, only Phe351, Phe174 and Gln179 are not conserved between ASIC1, ASIC2, ASIC3 and ASIC4 and Glu178, Thr215 and Glu354 display limited similarity ( Fig. 5 ). Together, these 6 ASIC1-specific residues provide 350 Å 2 of the total 860 Å 2 interaction surface between ASIC1 and PcTx1. Phe351 and Phe174 account for 155 Å 2 of the total binding surface. In ASIC2, ASIC3 and ASIC4, Phe351 is replaced by Ala, Leu and Ser, respectively, and mutating phenylalanine to leucine at this position in human ASIC1 abolishes PcTx1 binding ( Fig. 5c ) [15] . Phe174 is replaced by His173 in human ASIC1 that can retain the interaction with Arg27 of PcTx1 at low pH; however, Arg or Lys in ASIC2-4 introduce a positive charge and likely disturb the interaction with PcTx1 owing to repulsive forces. 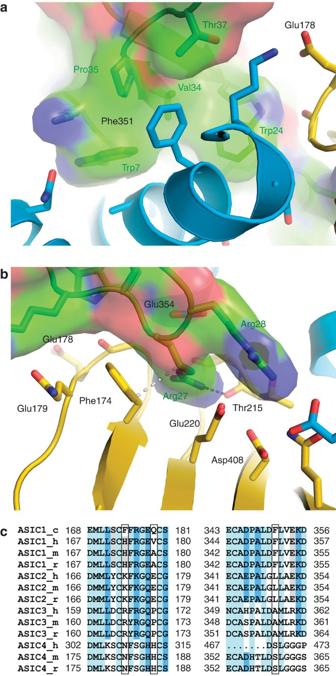Figure 5: Selectivity of PcTx1 for ASIC1 channels. Chicken ASIC1 residues of both the hydrophobic patch and the basic cluster that contribute the most to PcTx1 binding are not conserved among different ASICs. (a) The view on the ASIC1 helix 5 shows two subunits of ASIC1 (yellow and blue ribbon) and PcTx1 (transparent surface). The tight van der Waals interaction of Phe351 with the hydrophobic patch of PcTx1 is not retained in ASIC2, ASIC3 and ASIC4 channels that provide Leu, Ala or Ser residues instead. (b) Interactions between Phe174 and Arg27 of the basic cluster are important for PcTx1 binding. The interactions are retained at low pH if Phe174 is exchanged for His, as in human ASIC1 channels. In ASIC2, ASIC3 and ASIC4, Lys, Arg or Asn at position Phe174 introduce a positive charge and abolish binding. (c) Aperture of the Phe351, Phe174 and Gln179 regions in a sequence alignment of ASIC1 channel of various species. Light blue, dark blue and grey depict consensus regions; the rectangle highlights the position of the three ASIC1 residues crucial for selective PcTx1 binding. Figure 5: Selectivity of PcTx1 for ASIC1 channels. Chicken ASIC1 residues of both the hydrophobic patch and the basic cluster that contribute the most to PcTx1 binding are not conserved among different ASICs. ( a ) The view on the ASIC1 helix 5 shows two subunits of ASIC1 (yellow and blue ribbon) and PcTx1 (transparent surface). The tight van der Waals interaction of Phe351 with the hydrophobic patch of PcTx1 is not retained in ASIC2, ASIC3 and ASIC4 channels that provide Leu, Ala or Ser residues instead. ( b ) Interactions between Phe174 and Arg27 of the basic cluster are important for PcTx1 binding. The interactions are retained at low pH if Phe174 is exchanged for His, as in human ASIC1 channels. In ASIC2, ASIC3 and ASIC4, Lys, Arg or Asn at position Phe174 introduce a positive charge and abolish binding. ( c ) Aperture of the Phe351, Phe174 and Gln179 regions in a sequence alignment of ASIC1 channel of various species. Light blue, dark blue and grey depict consensus regions; the rectangle highlights the position of the three ASIC1 residues crucial for selective PcTx1 binding. Full size image The observed location of PcTx1 binding in the crystal structure is in very good agreement with the regions reported to be crucial for the binding to chimeric ASIC variants ( Supplementary Table S3 ) [22] ; however, the interactions differ significantly from those predicted in in silico docking studies [27] , [28] , [29] . A direct comparison reveals that none of the studies predicted more than one fourth of the interresidual interactions between PcTx1 and ASIC1 observed in the crystal structure ( Supplementary Table S4 ). Neither the charged interactions between the basic cluster arginines and the ASIC1 glutamates in the acidic pocket nor the intricate van der Waals interactions of the PcTx1 hydrophobic patch with helix 5 were correctly determined. The predicted models likely illustrate a non-physiological model of the complex as correctly expected [29] for the use of NMR structures with poorly defined regions for docking. Indeed, major differences are evident between the conformation of PcTx1 observed in the complex and the conformations of PcTx1 models used for docking ( Supplementary Fig. S5 ). The PcTx1–ASIC1 crystal structure provides an additional understanding for the effect that PcTx1 binding has for ion permeation and gating of ASIC1 channels. If compared with the ligand-free ASIC structures, a striking structural difference, a putative cation, is located near Glu80 and Glu417 of the occluded, central vestibule ( Fig. 4a ). This highlights the importance of the architecturally conserved central vestibule for ion conductance in trimeric sodium channels. In ASIC1, Leu78 separates the central vestibule that possibly functions as a cation reservoir from the extracellular vestibule that features the ion inlet windows [10] , [31] , [32] , whereas in P2X receptors, both vestibules are connected and accessible for ions that can enter the lateral fenestrations of the extracellular vestibule [31] . Strikingly, the only positively charged residue of the central vestibule, Arg370, is located right above the putative ion. As an arginine is also found at a similar location in P2X receptors (Arg321 (ref. 11 )), it might serve as a helper to expel ions from the cation reservoir towards the pore during channel opening. In the apo structure of ΔASIC1 (ref. 9 ), Glu80 and Glu417 form intrasubunit H-bonds and coordinate water molecules between the carboxylates of adjacent subunits. In the presence of PcTx1, the H-bond is disrupted and the three Glu417 carboxylate groups seem to coordinate the single ion right above Leu78 ( Fig. 4b ). Both Leu78 and Glu417 have been demonstrated to be crucial for ion permeation and gating [13] , [40] . Likely, the toxin-induced shift of the conformational equilibrium towards the closed state allows for the trapping of an ion in the cation reservoir. Its presence shows that the PcTx1 induced small conformational changes at the pH sensors, presumably the movement of the thumb helices 4 and 5, indirectly also affect the cation reservoir and the conducting pore. Because of its unique selectivity in modulating only ASIC1 channels, PcTx1 has been suggested to be of high therapeutic value but has not been reported as such. The complex structure can now serve as a starting template for the design of small molecules that maintain the selectivity of PcTx1 but achieve a better brain penetration. Such brain-penetrating small molecules would be the ideal pharmacological tools to further validate ASIC1 as a drug target and pave the way for the development of novel drugs against pain and various disorders of the central nervous system. Channel constructs and expression Four GenScript-optimized ASIC1 channel genes were cloned into modified pFastBac1 vectors and expressed in Spodoptera frugiperda (Sf9) cells. For the purification, SPR experiments and crystallization, chicken ΔASIC1(26-463) [9] , human ASIC1(1-467) and human ASIC1(25-464) constructs with an amino-terminal Kozak sequence, followed by a His 10 tag and either a PreScission or thrombin protease cleavage site, were used. Chicken ΔASIC1(26-463) proved to be the most promising construct for complex formation and crystallization of the desensitized-like conformation of ASIC1 (ref. 9 ). For the electrophysiological studies, we used full-length human ASIC1(1-528) with an N-terminal Kozak sequence followed by a His 10 -C9 tag. Baculovirus infection was performed with P1 virus at 0.1 % (v/v) virus concentration and Sf9 cell densities of 2×10 6 cells ml −1 in SF900II medium. Cells were cultured in a steel fermenter at 27 °C and collected ~55 h post-infection and stored at −80 °C. Electrophysiological experiments on human ASIC1(1-528) The pH dependence, PcTx1 and A-317567 inhibition of ASIC1-mediated currents were measured in manual whole-cell patch-clamp experiments using an EPC-9 amplifier. The holding potential was set to -80 mV. The extracellular saline contained 5 mM HEPES, 5 mM MES, 5 mM NaCl, 145 mM N -methyl- D -glucamine, 4 mM KCl, 1.2 mM CaCl 2 and 1 mM MgCl 2 . A HEPES/MES buffer mix was used to adjust the extracellular pH in a range from pH 5.7 to 7.4. The intracellular solution for the recording pipettes contained 10 mM HEPES(KOH) pH 7.2, 10 mM BAPTA, 130 mM KCl, 6 mM MgCl 2 and 5 mM Na 2 -ATP. To monitor the stability of channel function (run-down), a pH 6.0 control stimulus was repeatedly applied during the sequence of stimuli. Current amplitudes evoked by any test stimuli were visualized as a fraction of the control response amplitude estimated by interpolation between the next pH 6.0 stimuli. Purification Frozen Sf9 cell pellets were resuspended at 4 °C in a 1:8 ratio in a buffer containing 50 mM Tris(HCl) pH 8.0, 150 mM NaCl and protease inhibitor cocktail and disrupted by nitrogen cavitation at 4 °C, 30 bar pressure under stirring at 700 r.p.m.. Cell debris was removed by centrifugation at 488 g for 15 min and the supernatant centrifuged at 95,700 g for 35 min at 4 °C. After washing and ultracentrifugation, the membranes were resuspended in 50 mM Tris(HCl) pH 8.0, 150 mM NaCl and stored at −80 °C. Purified membranes corresponding to 100 g of cells were thawed and solubilized in 200 ml of a buffer containing 50 mM Tris(HCl) pH 8.0, 150 mM NaCl, 10 mM imidazole, 2% (w/v) n -dodecyl-β- D -maltopyranoside (DDM) under stirring for 60 min at 4 °C. The supernatant was isolated by centrifugation at 150,000 g for 20 min and purified using Talon Superflow IMAC resin at 4 °C. Washing and elution were performed in a buffer containing 50 mM Tris(HCl) pH 8.0, 150 mM NaCl, 0.05 % (w/v) DDM, either supplemented with 45 mM or 300 mM imidazole, respectively. The tag was removed with either PreScission protease at 4 °C or thrombin at room temperature for 1 h and, subsequently, 0.36 mg of synthetic, lyophilized PcTx1 (Peptanova) was dissolved directly in the protein solution. Excess PcTx1, protease and other buffer components were removed using a Superose 10/300 GL size exclusion column in 20 mM Tris(HCl) pH 8.0, 150 mM NaCl, 0.05% (w/v) DDM at 4 °C. For crystallization, the isolated, monodisperse protein preparation was concentrated to 2.7 mg ml −1 using an Amicon Ultra Ultracel centrifugal filter with a molecular weight cutoff of 100 kDa. For the SPR experiments, Talon-purified protein was purified, as described, without the addition of PcTx1 and directly biotinylated using EZ-Link NHS-Chromogenic-Biotin according to the Pierce instructions. Briefly, purified and cleaved ASIC1 protein was desalted on a HiPrep 26/10 column into phosphate-buffered saline containing 0.05% (w/v) DDM. The NHS-biotin reagent was added to ASIC at a 1:1 molar ratio and the reaction incubated at room temperature for 1 h. Excess, unincorporated label was removed by dialysis against a buffer containing 20 mM Tris(HCl) pH 8.0, 150 mM NaCl, 0.05 % (w/v) DDM and protein frozen and stored at −80 °C. Crystallization and structure determination For the chicken PcTx1-ΔASIC1 complex, crystals were produced by sitting drop vapour diffusion at 13 °C. Prism-shaped crystals were obtained by mixing protein 1:1 (v/v) with 100 mM sodium acetate pH 5.5, 3% glycerol, 3% 1,6-hexanediol, 11% PEG 6000. Crystals appeared within 3 days and matured within 1 week to a final size of 100 μm×25 μm×25 μm. The complex crystallized in the monoclinic space group C2 with one trimer per asymmetric unit. Crystals were collected directly from the crystal well supplemented with 15% glycerol for cryo-protection and flash frozen in liquid nitrogen. Diffraction data was collected to 3.0 Å resolution at a wavelength of 1.0000 Å using a PILATUS 6 M detector at the beamline X10SA of the Swiss Light Source (Paul Scherrer Institute, Villigen, Switzerland). The data was processed using XDS and scaled with SCALA. The complex structure was determined by molecular replacement with PHASER using the apo chicken ΔASIC1 structure as a start model. The difference electron density maps from the apo chicken ΔASIC1 solution ( Supplementary Methods ) were of sufficient quality to trace the toxin de novo , aided by the disulfide bonds of the cysteine knot as sequence markers ( Supplementary Fig. S6a, b ). Refinement was performed with PHENIX using NCS restraints for the extracellular domains of ASIC1 (residues 71-422) and PcTx1, except for Arg28 of the basic cluster. The quality of the final complex model was assessed using the Ramachandran plot in COOT (three outliers, 6.5% allowed), the rotamer analysis in COOT (6 outliers) and the Cβ deviations in PHENIX (maximum in the model: 0.16 Å) ( Supplementary Table S2 ). The toxin binding is unperturbed by crystal lattice contacts ( Supplementary Fig. 6c,d ). Figures were produced using Pymol. The structure coordinates have been deposited in the Protein Data Bank under the accession code ID 3S3X . SPR direct binding assays SPR experiments were performed with purified, biotinylated ASIC1 protein at 18 °C using streptavidin-coated SA biosensors and a Biacore 2000 instrument. To stabilize the immobilized ion channel, lipid detergent mixed micelles were applied [41] . For immobilization, ASIC1 protein diluted in a running buffer containing 20 mM sodium citrate pH 6.3, 300 mM NaCl, 0.05% DDM, 0.05% CHAPS, 0.01% CHS, 25 μM of a 7:3 (w/w) mixture of 1,2-dioleoyl- sn -glycero-3-phosphocholine:1,2-dioleoyl- sn -glycero-3-phospho- L -serine (DOPC:DOPS) to a final concentration of 6 μg ml −1 . Capturing was performed with a flow rate of 5 μl min −1 and free streptavidin was saturated by two 1 min injections of 1 μM biotin in running buffer. We aimed at rather low capturing levels of ASIC1 protein (741, 1068, 681 RU) to minimize toxin rebinding. Synthetic PcTx1 (PeptaNova) was titrated in running buffer with 5 concentrations in the range of 1.23 nM to 100 nM and a dilution factor of 3 in single-cycle kinetic mode in duplicate each at flow rates of 20 μl min −1 and 40 μl min −1 . Association and dissociation phases of the first 4 injections were monitored for 12 and 14 min, the highest PcTx1 concentration for 12 and 120 min. Blank kinetic cycles for all 5 injections of running buffer were run in parallel as a control. SPR response curves were analysed using the BIAevaluation software 3000 version 3.2 (Biacore AG). The sensograms were corrected for the response due to changes in the refractive index between running buffer and sample solutions by the subtraction of the corresponding curves from the reference channel 1. Kinetic data was extracted for all binding curves applying a one-to-one binding model fit on the experimental curves. Accession codes: Coordinates and structure factors have been deposited in the PDB database under accession codes 3S3W and 3S3X for apo and PcTx1-bound ASIC1, respectively. How to cite this article: Dawson, R.J.P. et al . Structure of the Acid-sensing ion channel 1 in complex with the gating modifier Psalmotoxin 1. Nat. Commun. 3:936 doi: 10.1038/ncomms1917 (2012).